A fast quantum interface between different spin qubit encodings Single-spin qubits in semiconductor quantum dots hold promise for universal quantum computation with demonstrations of a high single-qubit gate fidelity above 99.9% and two-qubit gates in conjunction with a long coherence time. However, initialization and readout of a qubit is orders of magnitude slower than control, which is detrimental for implementing measurement-based protocols such as error-correcting codes. In contrast, a singlet-triplet qubit, encoded in a two-spin subspace, has the virtue of fast readout with high fidelity. Here, we present a hybrid system which benefits from the different advantages of these two distinct spin-qubit implementations. A quantum interface between the two codes is realized by electrically tunable inter-qubit exchange coupling. We demonstrate a controlled-phase gate that acts within 5.5 ns, much faster than the measured dephasing time of 211 ns. The presented hybrid architecture will be useful to settle remaining key problems with building scalable spin-based quantum computers. Initialization, single-qubit and two-qubit gate operations, and measurements are fundamental elements for universal quantum computation [1] . Generally, they should all be fast and with high fidelity to reach the fault-tolerance thresholds [2] . So far, various encodings of spin qubits into one to three-spin subspaces have been developed in semiconductor quantum dots [3] , [4] , [5] , [6] , [7] , [8] , [9] , [10] , [11] , [12] , [13] , [14] , [15] . In particular, recent experiments demonstrated all of these elements including two-qubit logic gates for single-spin qubits proposed by Loss and DiVincenzo (LD qubits) and singlet-triplet (ST) qubits [6] , [7] , [8] , [14] . These qubits have different advantages depending on the gate operations, and combinations thereof can increase the performance of spin-based quantum computing. In LD qubits, the two-qubit gate is fast [6] , [7] as it relies on the exchange interaction between neighboring spins. In contrast, the two-qubit gate in ST qubits is much slower as it is mediated by a weak dipole coupling [14] . Concerning initialization and readout, however, the situation is the opposite: it is slow for LD qubits, relying on spin-selective tunneling to a lead [16] , [17] , while it is orders of magnitude faster in ST qubits relying on Pauli spin blockade [12] , [13] . Therefore, a fast and reliable interface between LD and ST qubits would allow for merging the advantages of both realizations. Here we present such an interface implementing a controlled-phase (CPHASE) gate between a LD qubit and a ST qubit in a quantum dot array [18] , [19] . The gate is based on the nearest neighbor exchange coupling and is performed in 5.5 ns. Even though we do not pursue benchmarking protocols here, the gate time being much shorter than the corresponding dephasing time (211 ns) indicates that the fidelity of this type of gates can be very high. Our results demonstrate that controlled coherent coupling of different types of gated spin qubits is feasible, and one can proceed to combining their advantages. Overall, our work pushes further the demonstrated scalability of spin qubits in quantum dot arrays. A LD qubit and a ST qubit formed in a triple quantum dot (TQD) A hybrid system comprising a LD qubit and a ST qubit is implemented in a linearly-coupled gate-defined TQD shown in Fig. 1a . The LD qubit (Q LD ) is formed in the left dot while the ST qubit (Q ST ) is hosted in the other two dots. We place a micro-magnet near the TQD to coherently and resonantly control Q LD via electric dipole spin resonance (EDSR) [20] , [21] , [22] , [23] , [26] . At the same time it makes the Zeeman energy difference between the center and right dots, \({\mathrm{\Delta }}E_{\mathrm{Z}}^{{\mathrm{ST}}}\) , much larger than their exchange coupling J ST , such that the eigenstates of Q ST become |↑↓〉 and |↓↑〉 rather than singlet |S〉 and triplet |T〉. We apply an external in-plane magnetic field B ext = 3.166 T to split the Q LD states by the Zeeman energy E Z as well as to separate polarized triplet states |↑↑〉 and |↓↓〉 from the Q ST computational states. The experiment is conducted in a dilution refrigerator with an electron temperature of approximately 120 mK. The qubits are manipulated in the (N L , N C , N R ) = (1,1,1) charge state while the (1,0,1) and (1,0,2) charge states are also used for initialization and readout (see Fig. 1b ). Here, N L(C,R) denotes the number of electrons inside the left (center, right) dot. Fig. 1 Hybrid system of a LD qubit and a ST qubit realized in a TQD. a False color scanning electron microscope image of a device identical to the one used in this study. The TQD is defined in a two-dimensional electron gas at the GaAs/AlGaAs heterointerface 100 nm below the surface. The upper single electron transistor is used for radiofrequency-detected charge sensing [24] , [25] . A MW with a frequency of 17.26 GHz is applied to the S gate to drive EDSR. b Stability diagram of the TQD obtained by differentiating the charge sensing signal V rf . c Hybrid system of a LD qubit and a ST qubit coupled by the exchange coupling J QQ . d Rabi oscillation of Q LD (rotation around x -axis) driven by EDSR with J QQ ~ 0 at point RL in Fig. 1b . The data is fitted to oscillations with a Gaussian decay of \(T_2^{{\mathrm{Rabi}}}\) = 199 ns. e Pulse sequence used to produce Fig. 1d showing gate voltages V PL and V PR applied to the PL and PR gates and a MW burst V MW . f Precession of Q ST (rotation around z -axis) with a frequency of f ST = 280 MHz due to \({\mathrm{\Delta }}E_{\mathrm{Z}}^{{\mathrm{ST}}}\) , taken at point E marked by the white circle in (1,1,1) in Fig. 1b , where J QQ and J ST ~ 0. The data follow the Gaussian decay with a decay time of 207 ns (see Supplementary Fig. 2a ) induced by the nuclear field fluctuations [29] . g Pulse sequence used to produce Fig. 1f Full size image We first independently measure the coherent time evolution of each qubit to calibrate the initialization, control, and readout. We quench the inter-qubit exchange coupling by largely detuning the energies of the (1,1,1) and (2,0,1) charge states. For Q LD , we observe Rabi oscillations [4] with a frequency f Rabi of up to 10 MHz (Fig. 1d ) as a function of the microwave (MW) burst time t MW , using the pulse sequence in Fig. 1e . For Q ST , we observe the precession between |S〉 and |T〉 (ST precession) (Fig. 1f ) as a function of the evolution time t e , using the pulse sequence in Fig. 1g (see Supplementary Note 2 for full control of Q ST ). We use a metastable state to measure Q ST with high fidelity [13] (projecting to |S〉 or |T〉) in the presence of large \({\mathrm{\Delta }}E_{\mathrm{Z}}^{{\mathrm{ST}}}\) with which the lifetime of |T〉 is short [27] . Calibration of the two-qubit coupling The two qubits are interfaced by exchange coupling J QQ between the left and center dots as illustrated in Fig. 1c . We operate the two-qubit system under the conditions of \(E_{\mathrm{Z}} \gg {\mathrm{\Delta }}E_{\mathrm{Z}}^{{\mathrm{ST}}},{\mathrm{\Delta }}E_{\mathrm{Z}}^{{\mathrm{QQ}}} \gg J^{{\mathrm{QQ}}} \gg J^{{\mathrm{ST}}}\) where \({\mathrm{\Delta }}E_{\mathrm{Z}}^{{\mathrm{QQ}}}\) is the Zeeman energy difference between the left and center dots. Then, the Hamiltonian of the system is 
    H = - E_Zσ̂_z^LD/2 - ΔE_Z^STσ̂_z^ST/2 + J^QQ(σ̂_z^LDσ̂_z^ST - 1)/4
 (1) where \(\hat \sigma _z^{{\mathrm{LD}}}\) and \(\hat \sigma _z^{{\mathrm{ST}}}\) are the Pauli z-operators of Q LD and Q ST , respectively [18] (Supplementary Note 3 ). The last term in Eq. ( 1 ) reflects the effect of the inter-qubit coupling J QQ : for states in which the spins in the left and center dots are antiparallel, the energy decreases by J QQ /2 (see Fig. 2a ). In the present work, we choose to operate Q LD as a control qubit and Q ST as a target, although these are exchangeable. With this interpretation, the ST precession frequency f ST depends on the state of Q LD, \(f_{\sigma _z^{{\mathrm{LD}}}}^{{\mathrm{ST}}} = \left( {{\mathrm{\Delta }}E_{\mathrm{Z}}^{{\mathrm{ST}}} - \sigma _z^{{\mathrm{LD}}}J^{{\mathrm{QQ}}}/2} \right)/h\) . Here \(\sigma _z^{{\mathrm{LD}}}\) represents |↑〉 or |↓〉 and +1 or −1 interchangeably. This means that while J QQ is turned on for the interaction time t int , Q ST accumulates the controlled-phase ϕ C = 2 πJ QQ t int / h , which provides the CPHASE gate (up to single-qubit phase gates; see Supplementary Note 7 ) in t int = h /2 J QQ . An important feature of this two-qubit gate is that it is intrinsically fast, scaling with J QQ / h which can be tuned up to ~100 MHz, and is limited only by the requirement \(J^{{\mathrm{QQ}}}/h \ll {\mathrm{\Delta }}E_{\mathrm{Z}}^{{\mathrm{QQ}}}/h \sim 500\,{\mathrm{MHz}}\) in our device. Fig. 2 ST qubit frequency controlled by the LD qubit. a Energy diagram of the two-qubit states for \(E_{\mathrm{Z}} \gg {\mathrm{\Delta }}E_{\mathrm{Z}}^{{\mathrm{ST}}},{\mathrm{\Delta }}E_{\mathrm{Z}}^{{\mathrm{QQ}}} \gg J^{{\mathrm{QQ}}}\) ( J ST = 0). The ST qubit frequency is equal to \({\mathrm{\Delta }}E_{\mathrm{Z}}^{{\mathrm{ST}}}\) for J QQ = 0, and shifts by ± J QQ /2 depending on the Q LD state for finite J QQ . b The quantum circuit for demonstrating the phase control of Q ST depending on Q LD . After preparing an arbitrary state of Q LD (stages A and B), we run modified stages from D to H (shown in the upper panel) 100 times with t int values ranging from 0.83 to 83 ns to observe the time evolution of Q ST without reinitializing or measuring Q LD . Stages A, B and C take 202 μs in total and the part from D to H is 7 μs long. c FFT spectra of f ST with different interaction points shown by the white corresponding symbol in Fig. 1b (traces offset for clarity). In addition to the frequency splitting due to J QQ , the center frequency of the two peaks shifts because \({\mathrm{\Delta }}E_{\mathrm{Z}}^{{\mathrm{ST}}}\) is also dependent on the interaction point (Methods). d Interaction point dependence of the ST qubit frequency splitting, i.e. the two-qubit coupling strength J QQ / h , fitted with the black model curve (see Supplementary Note 4 for the data extraction and fitting). e ST precession for the Q LD input state |↑〉 fitted with the Gaussian-decaying oscillations with a decay time of 72 ns. f ST precession for the Q LD input state |↓〉 with a fitting curve. The decay time is 75 ns. The total data acquisition time for e and f is 451 ms Full size image Before testing the two-qubit gate operations, we calibrate the inter-qubit coupling strength J QQ , and its tunability by gate voltages. The inter-qubit coupling in pulse stage F (Fig. 2b ) is controlled by the detuning energy between (2,0,1) and (1,1,1) charge states (one of the points denoted E in Fig. 1b ). To prevent leakage from the Q ST computational states, we switch J QQ on and off adiabatically with respect to \({\mathrm{\Delta }}E_{\mathrm{Z}}^{{\mathrm{QQ}}}\) by inserting voltage ramps to stage F with a total ramp time of t ramp = 24 ns (Fig. 2b ) [28] . The coherent precession of Q ST is measured by repeating the pulse stages from D to H without initializing, controlling and measuring Q LD , which makes Q LD a random mixture of |↑〉 and |↓〉. Figure 2c shows the FFT spectra of the precession measured for various interaction points indicated in Fig. 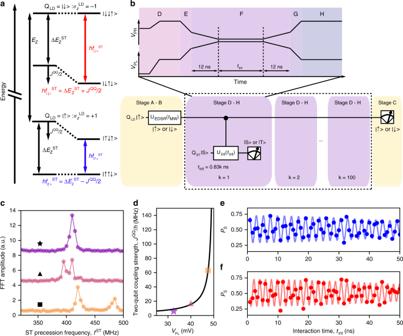Fig. 2 ST qubit frequency controlled by the LD qubit.aEnergy diagram of the two-qubit states for\(E_{\mathrm{Z}} \gg {\mathrm{\Delta }}E_{\mathrm{Z}}^{{\mathrm{ST}}},{\mathrm{\Delta }}E_{\mathrm{Z}}^{{\mathrm{QQ}}} \gg J^{{\mathrm{QQ}}}\)(JST= 0). The ST qubit frequency is equal to\({\mathrm{\Delta }}E_{\mathrm{Z}}^{{\mathrm{ST}}}\)forJQQ= 0, and shifts by ±JQQ/2 depending on the QLDstate for finiteJQQ.bThe quantum circuit for demonstrating the phase control of QSTdepending on QLD. After preparing an arbitrary state of QLD(stages A and B), we run modified stages from D to H (shown in the upper panel) 100 times withtintvalues ranging from 0.83 to 83 ns to observe the time evolution of QSTwithout reinitializing or measuring QLD. Stages A, B and C take 202 μs in total and the part from D to H is 7 μs long.cFFT spectra offSTwith different interaction points shown by the white corresponding symbol in Fig.1b(traces offset for clarity). In addition to the frequency splitting due toJQQ, the center frequency of the two peaks shifts because\({\mathrm{\Delta }}E_{\mathrm{Z}}^{{\mathrm{ST}}}\)is also dependent on the interaction point (Methods).dInteraction point dependence of the ST qubit frequency splitting, i.e. the two-qubit coupling strengthJQQ/h, fitted with the black model curve (see Supplementary Note4for the data extraction and fitting).eST precession for the QLDinput state |↑〉 fitted with the Gaussian-decaying oscillations with a decay time of 72 ns.fST precession for the QLDinput state |↓〉 with a fitting curve. The decay time is 75 ns. The total data acquisition time foreandfis 451 ms 1b . As we bring the interaction point closer to the boundary of (1,1,1) and (2,0,1), J QQ becomes larger and we start to see splitting of the spectral peaks into two. The separation of the two peaks is given by J QQ / h which can be controlled by the gate voltage as shown in Fig. 2d . We now demonstrate the controllability of the ST precession frequency by the input state of Q LD , the essence of a CPHASE gate. We use the quantum circuit shown in Fig. 2b , which combines the pulse sequences for independent characterization of Q LD and Q ST . Here we choose the interaction point such that J QQ / h = 90 MHz. By using either |↑〉 or |↓〉 as the Q LD initial state (the latter prepared by an EDSR π pulse), we observe the ST precessions as shown in Fig. 2e, f . The data fit well to Gaussian-decaying oscillations giving \(f_{| \uparrow \rangle}^{{\mathrm{ST}}} = 434 \pm 0.5\,{\mathrm{MHz}}\) and \(f_{| \downarrow \rangle}^{{\mathrm{ST}}} = 524 \pm 0.4\,{\mathrm{MHz}}\) [These are consistent with the values determined by Bayesian estimation discussed in Methods]. This demonstrates the control of the precession rate of Q ST by J QQ / h depending on the state of Q LD . Demonstration of a CPHASE gate To characterize the controlled-phase accumulated during the pulse stage F, we separate the phase of Q ST into controlled and single-qubit contributions as \(\phi _{\sigma _z^{{\mathrm{LD}}}} = - \pi \sigma _z^{{\mathrm{LD}}}J^{{\mathrm{QQ}}}\left( {t_{{\mathrm{int}}} + t_0} \right)/h\) and \(\phi ^{{\mathrm{ST}}} = 2\pi {\mathrm{\Delta }}E_{\mathrm{Z}}^{{\mathrm{ST}}}( {t_{{\mathrm{int}}} + t_{{\mathrm{ramp}}}} )/h + \phi _0\) , respectively. Here t 0 ( ≪ t ramp ) represents the effective time for switching on and off J QQ (Supplementary Note 5 ). A phase offset ϕ 0 denotes the correction accounting for nonuniform \({\mathrm{\Delta }}E_{\mathrm{Z}}^{{\mathrm{ST}}}\) during the ramp (Supplementary Note 5 ). Then the probability of finding the final state of Q ST in singlet is modeled as 
    P_S,model = acos( ϕ _σ _z^LD + ϕ ^ST)exp(  - (t_int/T_2^ ∗ ))^2 + b
 (2) where a , b and \(T_2^ \ast\) represent the values of amplitude, mean and the dephasing time of the ST precession, respectively. We use maximum likelihood estimation (MLE) combined with Bayesian estimation [29] , [30] to fit all variables in Eq. 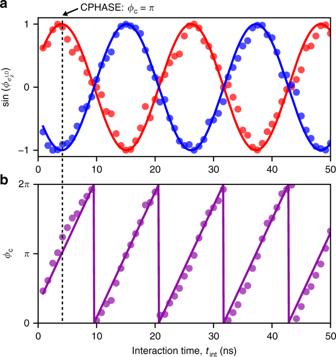Fig. 3 Controlled-phase evolution.aInteraction timetintdependence of\(\phi _{\sigma _z^{{\mathrm{LD}}}}\)controlled by QLD. The blue and red data are for QLD= |↑〉 and |↓〉, respectively. The solid curves are sin(πJQQ(tint+t0)/h) (red) and sin(−πJQQ(tint+t0)/h) (blue) where the values ofJQQandt0are obtained in the MLE. The curves are consistent with the data as expected.bControlled-phaseϕC=ϕ|↓〉−ϕ|↑〉extracted from Fig.3a. Including the initial phase accumulated during gate voltage ramps at stage F,ϕCreachesπfirst attint= 4.0 ns and increases byπin every 5.5 ns afterwards 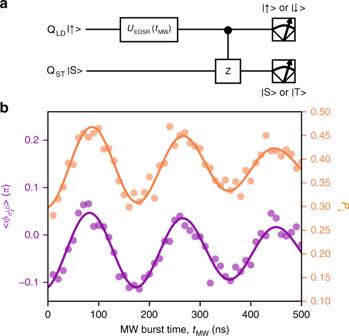Fig. 4 Demonstration of the controlled-phase gate for arbitrary control qubit states.aThe circuit for CPHASE gate demonstration. Heretintis fixed at 4.2 ns whereϕC≈π(Fig.3b).btMWdependence of the spin-down probability of QLD,P↓(yellow) and the averaged\(\phi _{\sigma _z^{{\mathrm{LD}}}}\),\(\left\langle \phi _{\sigma _z^{{\mathrm{LD}}}} \right\rangle\)(purple) obtained by the circuit shown in Fig.4a.\(\left\langle \phi _{\sigma _z^{{\mathrm{LD}}}} \right\rangle\)\(\left( { = - \pi \langle \sigma _z^{{\mathrm{LD}}} \rangle /2} \right)\)is expected to be proportional toP↓. We see\(\left\langle \phi _{\sigma _z^{{\mathrm{LD}}}} \right\rangle\)oscillates depending on the input QLDstate. The oscillation visibility of\(\left\langle \phi _{\sigma _z^{{\mathrm{LD}}}} \right\rangle\)is most probably limited by low preparation fidelity of the input QLDstate as the visibility of the oscillation inP↓is also low (see Methods) 2, that are \(a,b,t_0,J^{{\mathrm{QQ}}},T_2^ \ast ,\phi _0\) , and \({\mathrm{\Delta }}E_{\mathrm{Z}}^{{\mathrm{ST}}}\) , from the data (Methods). This allows us to extract the t int dependence of \(\phi _{\sigma _z^{{\mathrm{LD}}}}\) (Fig. 3a ) (Methods) and consequently ϕ C = ϕ | ↓〉 − ϕ |↑〉 (Fig. 3b ). It evolves with t int in the frequency of J QQ / h = 90 MHz, indicating that the CPHASE gate time can be as short as h /2 J QQ = 5.5 ns (up to single-qubit phase). On the other hand, \(T_2^ \ast\) obtained in the MLE is 211 ns, much longer than what is observed in Fig. 2e, f because the shorter data acquisition time used here cuts off the low-frequency component of the noise spectrum [29] . We note that this \(T_2^ \ast\) is that for the two-qubit gate while J QQ is turned on [8] , and therefore it is likely to be dominated by charge noise rather than the nuclear field fluctuation (Supplementary Note 6 ). The ratio \(2J^{{\mathrm{QQ}}}T_2^ \ast /h\) suggests that 38 CPHASE operations would be possible within the two-qubit dephasing time. We anticipate that this ratio can be further enhanced by adopting approaches used to reduce the sensitivity to charge noise in exchange gates such as symmetric operation [31] , [32] and operation in an enhanced field gradient [33] . Fig. 3 Controlled-phase evolution. a Interaction time t int dependence of \(\phi _{\sigma _z^{{\mathrm{LD}}}}\) controlled by Q LD . The blue and red data are for Q LD = |↑〉 and |↓〉, respectively. The solid curves are sin( πJ QQ ( t int + t 0 )/ h ) (red) and sin(− πJ QQ ( t int + t 0 )/ h ) (blue) where the values of J QQ and t 0 are obtained in the MLE. The curves are consistent with the data as expected. b Controlled-phase ϕ C = ϕ |↓〉 − ϕ |↑〉 extracted from Fig. 3a . Including the initial phase accumulated during gate voltage ramps at stage F, ϕ C reaches π first at t int = 4.0 ns and increases by π in every 5.5 ns afterwards Full size image Finally we show that the CPHASE gate operates correctly for arbitrary Q LD input states. We implement the circuit shown in Fig. 4a in which t int is fixed to yield ϕ C = π , while a coherent initial Q LD state with an arbitrary \(\sigma _z^{{\mathrm{LD}}}\) is prepared by EDSR. We extract the averaged \(\phi _{\sigma _z^{{\mathrm{LD}}}}\) , \(\left\langle \phi _{\sigma _z^{{\mathrm{LD}}}} \right\rangle\) by Bayesian estimation [29] , [30] , which shows an oscillation as a function of t MW in agreement with the Rabi oscillation measured independently by reading out Q LD at stage C as shown in Fig. 4b (see Methods for the estimation procedure and the origin of the low visibility, i.e., \({\mathrm{max}}| {\langle {\phi _{\sigma _z^{{\mathrm{LD}}}}} \rangle } | < \pi /2\) ). These results clearly demonstrate the CPHASE gate functioning for an arbitrary Q LD input state. Fig. 4 Demonstration of the controlled-phase gate for arbitrary control qubit states. a The circuit for CPHASE gate demonstration. Here t int is fixed at 4.2 ns where ϕ C ≈ π (Fig. 3b ). b t MW dependence of the spin-down probability of Q LD , P ↓ (yellow) and the averaged \(\phi _{\sigma _z^{{\mathrm{LD}}}}\) , \(\left\langle \phi _{\sigma _z^{{\mathrm{LD}}}} \right\rangle\) (purple) obtained by the circuit shown in Fig. 4a . \(\left\langle \phi _{\sigma _z^{{\mathrm{LD}}}} \right\rangle\) \(\left( { = - \pi \langle \sigma _z^{{\mathrm{LD}}} \rangle /2} \right)\) is expected to be proportional to P ↓ . We see \(\left\langle \phi _{\sigma _z^{{\mathrm{LD}}}} \right\rangle\) oscillates depending on the input Q LD state. The oscillation visibility of \(\left\langle \phi _{\sigma _z^{{\mathrm{LD}}}} \right\rangle\) is most probably limited by low preparation fidelity of the input Q LD state as the visibility of the oscillation in P ↓ is also low (see Methods) Full size image In summary, we have realized a fast quantum interface between a LD qubit and a ST qubit using a TQD. The CPHASE gate between these qubits is performed in 5.5 ns, much faster than its dephasing time of 211 ns and those ratio (~38) would be high enough to provide a high-fidelity CPHASE gate (Supplementary Note 8 ). Optimizing the magnet design to enhance the field gradient would allow even faster gate time beyond GHz with larger J QQ . At the same time, this technique is directly applicable to Si-based devices with much better single-qubit coherence [5] , [6] , [7] , [8] , [9] . Our results suggest that the performance of certain quantum computational tasks can be enhanced by adopting different kinds of qubits for different roles. For instance, LD qubits can be used for high-fidelity control and long memory and the ST qubit for fast initialization and readout. This combination is ideal for example, the surface code quantum error correction where a data qubit must maintain the coherence while a syndrome qubit must be measured quickly [34] . Furthermore, the fast (~100 ns [25] ) ST qubit readout will allow the read out of a LD qubit in a quantum-non-demolition manner [35] with a speed three orders of magnitude faster than a typical energy-selective tunneling measurement [16] , [17] . Viewed from the opposite side, we envisage coupling two ST qubits through an intermediate LD qubit, which would boost the two ST qubit gate speed by orders of magnitude compared to the demonstrated capacitive coupling scheme [14] . In addition, our results experimentally support the concept of the theoretical proposal of a fast two-qubit gate between two ST qubits based on direct exchange [36] which shares the same working principle as our two-qubit gate. Our approach will further push the demonstrated scalability of spin qubits in quantum dot arrays beyond the conventional framework based on a unique spin-qubit encoding. Device design Our device was fabricated on a GaAs/Al 0.3 Ga 0.7 As heterostructure wafer having a two-dimensional electron gas 100 nm below the surface, grown by molecular beam epitaxy on a semi-insulating (100) GaAs substrate. The electron density n and mobility μ at a temperature of 4.2 K are n = 3.21 × 10 15 m −2 and μ = 86.5 m 2 V −1 s −1 in the dark, respectively. We deposited Ti/Au gate electrodes to define the TQD and the charge sensing single electron transistor. A piece of Co metal (micro-magnet, MM) is directly placed on the surface of the wafer to provide a local magnetic field gradient in addition to the external magnetic field applied in-plane (along z ). The MM geometry is designed based on the numerical simulations of the local magnetic field [23] . The field property is essentially characterized by the two parameters [23] : d B x /d z at the position of each dot and the difference in B z between the neighboring dots, Δ B z (see Fig. 1a for the definition of the x and z axes). d B x /d z determines the spin rotation speed by EDSR and is as large as ~1 mT nm −1 at the left dot (Supplementary Fig. 5a ) allowing fast control of Q LD ( f Rabi > 10 MHz) [20] , [23] . At the same time Δ B z between the left and center dots, \({\mathrm{\Delta }}B_z^{{\mathrm{LC}}}\) , is designed to be ~60 mT (Supplementary Fig. 5b ) to guarantee the selective EDSR control of Q LD without rotating the spin in the center dot [20] , [23] . Furthermore, Δ B z between the center and right dots, \({\mathrm{\Delta }}B_z^{{\mathrm{CR}}}\) , is designed to be ~40 mT (Supplementary Fig. 5b ) to make the eigenstates of Q ST |↑↓〉 and |↓↑〉 rather than |S〉 and |T〉 by satisfying \({\mathrm{\Delta }}E_{\mathrm{Z}}^{{\mathrm{ST}}} \gg J^{{\mathrm{ST}}}\) . Note that \({\mathrm{\Delta }}E_{\mathrm{Z}}^{{\mathrm{ST}}} = |g|\mu _{\mathrm{B}}{\mathrm{\Delta }}B_z^{{\mathrm{CR}}}\) where g ~ −0.4 and μ B are the electron g -factor and Bohr magneton, respectively. From the design we expect a large variation of \({\mathrm{\Delta }}B_z^{{\mathrm{CR}}}\) when the electron in the center dot is displaced by the electric field. Indeed, we observe a strong influence of the gate voltages on \({\mathrm{\Delta }}B_z^{{\mathrm{CR}}}\) , which reaches ~100 mT \(\left( {{\mathrm{\Delta }}E_{\mathrm{Z}}^{{\mathrm{ST}}}/h \sim 500\,{\mathrm{MHz}}} \right)\) in the configuration chosen for the two-qubit gate experiment. Estimation of the ST precession parameters Here we describe the estimation of the ST precession parameters in Eq. 2 under the influence of a fluctuating single-qubit phase of Q ST . Out of the parameters involved, \(\phi _{\sigma _z^{{\mathrm{LD}}}}\) is the only parameter assumed to be Q LD state-dependent, and the rest is classified into two types. One is the pulse-cycle-independent parameters, \(a,b,J^{{\mathrm{QQ}}},T_2^ \ast\) and t 0 which is constant during the experiment, and the other is the pulse-cycle-dependent parameters, \(\sigma _z^{{\mathrm{LD}}},{\mathrm{\Delta }}E_{\mathrm{Z}}^{{\mathrm{ST}}}\) and ϕ 0 , which can change cycle by cycle. Each pulse cycle consists of pulse stages from A to C as shown in Fig. 2b . 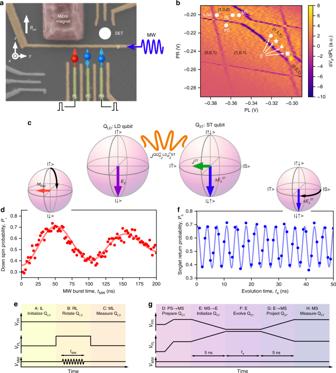We run the pulse cycle consecutively with a MW frequency fixed at 17.26 GHz and collect the data while Q LD drifts between on-resonances and off-resonances with the MW burst due to the nuclear field fluctuation. To decrease the uncertainty of the estimated parameters, we choose the cycles during which the spin flip of Q LD is unlikely in the following manner. The cycles throughout which Q LD is likely to be |↓〉 are post-selected by the condition that Q LD is on-resonance (i.e., Rabi oscillation of Q LD is observed in ensemble-averaged data from nearby cycles) and the final state of Q LD is measured to be |↓〉 at pulse stage C. Similarly, the cycles for Q LD = |↑〉 are post-selected by the condition that Q LD is off-resonance and the final state of Q LD is measured to be |↑〉. Fig. 1 Hybrid system of a LD qubit and a ST qubit realized in a TQD.aFalse color scanning electron microscope image of a device identical to the one used in this study. The TQD is defined in a two-dimensional electron gas at the GaAs/AlGaAs heterointerface 100 nm below the surface. The upper single electron transistor is used for radiofrequency-detected charge sensing24,25. A MW with a frequency of 17.26 GHz is applied to the S gate to drive EDSR.bStability diagram of the TQD obtained by differentiating the charge sensing signalVrf.cHybrid system of a LD qubit and a ST qubit coupled by the exchange couplingJQQ.dRabi oscillation of QLD(rotation aroundx-axis) driven by EDSR withJQQ~ 0 at point RL in Fig.1b. The data is fitted to oscillations with a Gaussian decay of\(T_2^{{\mathrm{Rabi}}}\)= 199 ns.ePulse sequence used to produce Fig.1dshowing gate voltagesVPLandVPRapplied to the PL and PR gates and a MW burstVMW.fPrecession of QST(rotation aroundz-axis) with a frequency offST= 280 MHz due to\({\mathrm{\Delta }}E_{\mathrm{Z}}^{{\mathrm{ST}}}\), taken at point E marked by the white circle in (1,1,1) in Fig.1b, whereJQQandJST~ 0. The data follow the Gaussian decay with a decay time of 207 ns (see Supplementary Fig.2a) induced by the nuclear field fluctuations29.gPulse sequence used to produce Fig.1f The data structure and the index definitions for MLE are summarized in Supplementary Table 1 . k is the index of the interaction time such that t int = 0.83 × k ns with k ranging from 1 to 100. m is the pulse-cycle index ranging from 1 (2001) to 2000 (4000) for Q LD prepared in |↑〉 (|↓〉). The estimation procedure is the following. From all the readout results of Q ST (stage H) obtained in the cycles, we first estimate the five pulse-cycle-independent parameters by MLE. Note that J QQ may have a small pulse-cycle-dependent component due to charge noise but this effect is captured as additional fluctuation in \({\mathrm{\Delta }}E_{\mathrm{Z}}^{{\mathrm{ST}}}\) and ϕ 0 in our model. We apply MLE to 100 × 4000 readout results of Q ST , \(r_m^k = 1\) (0) for Q ST = |S〉 (|T〉). To this end, we first introduce the likelihood P m defined in the eight dimensional parameter space as 
    P_m( a,b,t_0,J^QQ,T_2^ ∗ ,σ _z^LD,ϕ _0,ΔE_Z^ST) = ∏_k = 1^100( r_m^kP_S,model + (1 - r_m^k)(1 - P_S,model))
 (3) where P S,model is defined in Eq. (2). We calculate P m on a discretized space within a chosen parameter range (Supplementary Table 2 ) using a single cycle data. Then we obtain P m for the target five parameters as a marginal distribution by tracing out the pulse-cycle-dependent parameters, 
    P_m( a,b,t_0,J^QQ,T_2^ ∗) = ∑_σ _z^LD∑_ϕ _0∑_ΔE_Z^ST P_m( a,b,t_0,J^QQ,T_2^ ∗ ,σ _z^LD,ϕ _0,ΔE_Z^ST). (4) Repeating this process for all pulse cycles, we obtain the likelihood P as 
    P( a,b,t_0,J^QQ,T_2^ ∗) = ∏_m P_m( a,b,t_0,J^QQ,T_2^ ∗). (5) We choose the maximum of P as the estimator for a , b , t 0 , J QQ and \(T_2^ \ast\) , obtaining a = 0.218 ± 0.005, b = 0.511 ± 0.003, t 0 = 1.53 ± 0.17 ns, J QQ / h = 90.2 ± 0.3 MHz, \(T_2^ \ast = 211 \pm 37\) ns. Once these values are fixed, we estimate the pulse-cycle-dependent parameters, \(\sigma _z^{{\mathrm{LD}}},\phi _0\) and \({\mathrm{\Delta }}E_{\mathrm{Z}}^{{\mathrm{ST}}}\) , for each cycle m . Note that \(\sigma _z^{{\mathrm{LD}}}\) could be prepared deterministically if the state preparation of Q LD were ideal, but here we treat it as one of the parameters to be estimated because of a finite error in the Q LD state preparation. We again evaluate the likelihood \(P_m\left( {\sigma _z^{{\mathrm{LD}}},\phi _0,{\mathrm{\Delta }}E_{\mathrm{Z}}^{{\mathrm{ST}}}} \right)\) defined in a discretized three dimensional space of its parameters using Eq. 3 and find their values that maximize the likelihood. Based on the values of \(a,b,T_2^ \ast\) and ϕ ST determined above, we can directly estimate \(\phi _{\sigma _z^{{\mathrm{LD}}}}\) controlled by Q LD for each t int without presumptions on the value of J QQ . To this end, we search for the parameter \(\phi _{\sigma _z^{{\mathrm{LD}}}}\) that maximizes the likelihood 
    P^k( ϕ _σ _z^LD) = ∏_m ( r_m^kP_S,model + ( 1 - r_m^k)( 1 - P_S,model)). (6) The obtained estimators for ϕ |↓〉 and ϕ |↑〉 are consistent with the expected values ± πJ QQ ( t int + t 0 )/ h calculated from J QQ / h and t 0 found above (see Fig. 3a ). The ensemble-averaged phase \(\left\langle {\phi _{\sigma _z^{{\mathrm{LD}}}}} \right\rangle\) is obtained based on a similar estimation protocol. Here we estimate \(\phi _{\sigma _z^{{\mathrm{LD}}}}\) for each m with fixed k = 5 ( t int = 4.2 ns) to yield ϕ C ≈ π from the likelihood \(P_m^{k = 5} = r_m^{k = 5}P_{{\mathrm{S}},{\mathrm{model}}} + \left( {1 - r_m^{k = 5}} \right)\left( {1 - P_{{\mathrm{S}},{\mathrm{model}}}} \right)\) and then take the average of the estimated values for 800 pulse cycles. The oscillation visibility of \(\left\langle {\phi _{\sigma _z^{{\mathrm{LD}}}}} \right\rangle\) in Fig. 4b is limited by three factors, low preparation fidelity of the input Q LD state, estimation error of \(\phi _{\sigma _z^{{\mathrm{LD}}}}\) and CPHASE gate error. The first contribution is likely to be dominant as the visibility of the oscillation in P ↓ is correspondingly low. Note that the effect of those errors is not visible in Fig. 3 because the most likely values of \(\phi _{\sigma _z^{{\mathrm{LD}}}}\) are plotted.